Pathway and network analysis of more than 2500 whole cancer genomes The catalog of cancer driver mutations in protein-coding genes has greatly expanded in the past decade. However, non-coding cancer driver mutations are less well-characterized and only a handful of recurrent non-coding mutations, most notably TERT promoter mutations, have been reported. Here, as part of the ICGC/TCGA Pan-Cancer Analysis of Whole Genomes (PCAWG) Consortium, which aggregated whole genome sequencing data from 2658 cancer across 38 tumor types, we perform multi-faceted pathway and network analyses of non-coding mutations across 2583 whole cancer genomes from 27 tumor types compiled by the ICGC/TCGA PCAWG project that was motivated by the success of pathway and network analyses in prioritizing rare mutations in protein-coding genes. While few non-coding genomic elements are recurrently mutated in this cohort, we identify 93 genes harboring non-coding mutations that cluster into several modules of interacting proteins. Among these are promoter mutations associated with reduced mRNA expression in TP53 , TLE4 , and TCF4 . We find that biological processes had variable proportions of coding and non-coding mutations, with chromatin remodeling and proliferation pathways altered primarily by coding mutations, while developmental pathways, including Wnt and Notch, altered by both coding and non-coding mutations. RNA splicing is primarily altered by non-coding mutations in this cohort, and samples containing non-coding mutations in well-known RNA splicing factors exhibit similar gene expression signatures as samples with coding mutations in these genes. These analyses contribute a new repertoire of possible cancer genes and mechanisms that are altered by non-coding mutations and offer insights into additional cancer vulnerabilities that can be investigated for potential therapeutic treatments. Over the past decade, cancer genome sequencing efforts such as The Cancer Genome Atlas (TCGA) have identified millions of somatic aberrations; however, the annotation and interpretation of these aberrations remain a major challenge [1] . Specifically, while some somatic aberrations occur frequently in specific cancer types, there is a “long tail” of rare aberrations that are difficult to distinguish from random passenger aberrations in modestly sized patient cohorts [2] , [3] . In many cancers, a significant proportion of patients do not have known driver mutations in protein-coding regions [4] , suggesting that additional driver mutations remain undiscovered. The vast majority of known driver mutations affect protein-coding regions. Only a few recurrent non-coding driver mutations, most notably mutations in the TERT promoter [5] , [6] , have been identified. In other studies, a genome-wide analysis has identified recurrent mutations in several regulatory elements, and expression quantitative trait loci (eQTLs) analysis has identified non-coding somatic mutations that correlate with gene expression changes in some cancer types [7] . Cancer driver mutations unlock oncogenic properties of cells by altering the activity of hallmark pathways [8] . Accordingly, cancer genes have been shown to cluster in a small number of cellular pathways and interacting subnetworks [3] , [9] . Consequently, pathway and network analysis has proven useful for implicating infrequently mutated genes as cancer genes based on their pathway membership and physical or regulatory interactions with recurrently mutated genes [10] , [11] , [12] , [13] , [14] . However, the interactions between coding and non-coding driver mutations in known or novel pathways have not yet been systematically explored. As part of the Pan-Cancer Analysis of Whole Genomes (PCAWG) project of the International Cancer Genome Consortium (ICGC) [15] , we performed pathway and network analysis of coding and non-coding somatic mutations from 2583 tumors from 27 tumor types. The PCAWG consortium curated whole-genome sequencing data from a total of 2658 cancers across 38 tumor types. In the marker paper [15] , this work provided the largest collection of uniformly processed cancer whole genomes to date with germline and somatic variants from reanalyzed sequencing data aligned to the human genome (reference build hs37d5) using standardized and highly accurate pipelines. Recent work from the PCAWG project of the ICGC reveals few recurrent non-coding drivers in analyses of individual genes and regulatory regions [16] . Here, we employ seven distinct pathways and network analysis methods and derive consensus sets of pathway-implicated driver (PID) genes from the predictions of these methods. Specifically, we identify a consensus set of 93 high-confidence pathway-implicated driver genes using non-coding variants (PID-N) and a consensus set of 87 pathway-implicated driver genes using coding variants (PID-C). Both sets of PID genes, particularly the PID-N set, contain rarely mutated genes that interact with well-known cancer genes, but were not identified as significantly mutated by single gene tests [16] . In total, 121 novel PID-N and PID-C genes are revealed as promising candidates, expanding the landscape of driver mutations in cancer. We examined the relative contributions of coding and non-coding mutations in altering biological processes, finding that while chromatin remodeling and some well-known signaling and proliferation pathways are altered primarily by coding mutations, other important cancer pathways, including developmental pathways, such as Wnt and Notch, are altered by both coding and non-coding mutations in PID genes. Intriguingly, we find many non-coding mutations in PID-N genes with roles in RNA splicing, and samples with these non-coding mutations exhibit similar gene expression signatures as samples with well-known coding mutations in RNA splicing factors. Our analysis demonstrates that somatic non-coding mutations in untranslated and in cis regulatory regions constitute a complementary set of genetic perturbations with respect to coding mutations, affect several biological pathways and molecular interaction networks, and should be further investigated for their role in the onset and progression of cancer. The long tail of coding and non-coding driver mutations We analyzed the genes targeted by single-nucleotide variants (SNVs) and short insertions and deletions (indels) identified by whole-genome sequencing in the 2538 ICGC PCAWG tumor samples from 27 tumor types. Our pathway and network analyses focused on a subset of 2252 tumors that excluded melanomas and lymphomas due to their atypical distributions of mutations in regulatory regions [17] . We utilized the pan-cancer driver p -values of single protein-coding and non-coding elements from the PCAWG Drivers and Functional Interpretation Working Group analysis [16] , including exons, promoters, untranslated regions (5′ UTR and 3′ UTR), and enhancers. This analysis integrates predictions from 16 driver discovery methods, resulting in consensus driver p -values for coding and non-coding elements; see ref. [16] for further details. The p -values of individual genes and non-coding elements indicate their statistical significance as drivers, according to diverse methods that account for positive selection, functional impact of mutations, regional mutation rates, and mutational processes and signatures [16] . Among protein-coding driver p -values of the pan-cancer cohort, 75 genes were statistically significant (FDR < 0.1; Supplementary Fig. 1 ) and an additional 7 genes were observed at near-significant levels (0.1 ≤ FDR < 0.25). These numbers are consistent with previous reports of a “long tail” of driver genes with few highly mutated genes and many genes with infrequent mutations across cancer types [2] , [18] . Non-coding mutations exhibit a similar long-tail distribution with even fewer significant genes (eight genes at FDR < 0.1 and two genes at 0.1 ≤ FDR < 0.25). No single gene has both significant or near-significant coding and non-coding driver p -values (FDR < 0.25), suggesting that non-coding mutations target a complementary set of genes as coding mutations. Earlier studies have demonstrated that proteins harboring coding driver mutations interact with each other in molecular pathways and networks significantly more frequently than expected by chance [2] , [3] , [9] , [10] , [11] , [13] . We observed significant numbers of interactions between both significantly mutated coding and/or non-coding elements, suggesting that the pathway and network methods may be useful in prioritizing rare driver events that are not significant by single-element analyses (Supplementary Fig. 2 ; Coding and non-coding mutations cluster on networks in Supplementary file). Pathway and network analysis of potential driver mutations We performed a comprehensive pathway and network analysis of cancer drivers using the single-element driver p -values computed by the PCAWG Drivers and Functional Interpretation Working Group [16] as input. We applied seven distinct pathways and network methods (ActivePathways [19] , CanIsoNet [20] , Hierarchical HotNet [21] , a hypergeometric analysis (Vazquez), an induced subnetwork analysis (Reyna and Raphael, in preparation), NBDI [22] , and SSA-ME [23] ) that each leverage information from molecular pathways or protein interaction networks (Fig. 1 , Methods section) to amplify weak signals in the single-element analysis. All methods were calibrated on randomized data (Pathway and network methods in Supplementary file). Fig. 1: Overview of the pathway and network analysis approach. Coding, non-coding, and combined gene scores were derived for each gene by aggregating driver p -values from the PCAWG driver predictions in individual elements, including annotated coding and non-coding elements (promoter, 5′ UTR, 3′ UTR, and enhancer). These gene scores were input to five network analysis algorithms (CanIsoNet [20] , Hierarchical HotNet [21] , an induced subnetwork analysis (Reyna and Raphael, in preparation), NBDI [22] , and SSA-ME [23] ), which utilize multiple protein–protein interaction networks, and to two pathway analysis algorithms (ActivePathways [19] and a hypergeometric analysis (Vazquez)), which utilize multiple pathway/gene-set databases. We defined a non-coding value-added (NCVA) procedure to determine genes whose non-coding scores contribute significantly to the results of the combined coding and non-coding analysis, where NCVA results for a method augment its results on non-coding data. We defined a consensus procedure to combine significant pathways and networks identified by these seven algorithms. The 87 pathway-implicated driver genes with coding variants (PID-C) are the set of genes reported by a majority (≥4/7) of methods on the coding data. The 93 pathway-implicated driver genes with non-coding variants (PID-N) are the set of genes reported by a majority of methods on non-coding data or in their NCVA results. Only five genes ( CTNNB1 , DDX3X , SF3B1 , TGFBR2 , and TP53 ) are both PID-C and PID-N genes. Full size image Since the prioritization of non-coding somatic mutations in cancer is not yet a solved problem, it was difficult to know in advance which analysis methodologies, if any, would be best suited to distinguish drivers from passengers by aggregating weak signals across pathways or networks. Thus, we formed a consensus of multiple methods, following the “wisdom of crowds” ensemble approach of machine learning [24] to improve the specificity of the results. We included methods that used different sources of pathway or network information and different prioritization criteria (see Supplementary Data 1 for a complete list). Each method nominated genes, and consensus sets of genes with possible coding and non-coding driver mutations were defined as the genes found by at least four of the seven methods (Supplementary Data 2 – 5 ). We use the term pathway-implicated driver (PID) genes to describe these candidate driver genes. One potential concern with a consensus procedure is that the results may be dominated by a few highly correlated methods. Our pathway or network analysis methods use varied sources of prior knowledge (i.e., pathway databases or interaction networks), and input data (e.g., driver p -values, point mutations, and/or gene expression), and rely on different techniques to integrate these data sources. We found only a modest overlap between the output of the seven methods (Method results comparison and Consensus procedure in Supplementary file; Supplementary Data 6 – 8 ), suggesting a non-uniform weighting of the consensus to mitigate the influence of redundant methods was not necessary. Using coding mutations alone, we identify a set of 87 pathway-implicated driver genes with coding variants (PID-C genes). The 87 PID-C genes (Supplementary Data 2 , Supplementary Fig. 6a ) include 68 previously identified cancer genes as catalogued by the COSMIC Cancer Gene Census (CGC) database (v83, 699 genes from Tier 1 and Tier 2) [25] (2.98 genes expected; Fisher′s exact test p = 3.57 × 10 −83 ; Fig. 2a, c ; Supplementary Fig. 7a ). The PID-C genes have significantly higher coding gene scores than non-PID-C genes (rank-sum test p = 1.72 × 10 −58 ; median rank 48 of PID-C genes), and each of the 87 PID-C genes improves the score of its network neighborhood (19.7 genes expected; p < 10 −6 ; Supplementary Data 9 ). This network neighborhood analysis shows that PID-C genes are not implicated solely by their network neighbors [14] , but themselves contribute significantly to their discovery by the pathway and network methods. The 87 PID-C genes also include 31 genes that are not statistically significant (FDR > 0.1) in the PCAWG Drivers and Functional Interpretation Working Group analysis; Fig. 2a, c ; Supplementary Figs. 8a , 9 ), illustrating that the network neighborhoods can nominate genes with infrequent mutations, i.e., those in the “long tail”, as possible driver genes. Interestingly, 13 of these 31 genes with FDR > 0.1 are also known drivers according to the CGC database (3.0 genes expected; Fisher’s exact test p = 2.1 × 10 −14 ). Thus, the consensus pathway and network analysis recovers many known protein-coding driver mutations and identifies additional possible drivers that are infrequently mutated and thus remain below the statistical significance threshold of gene-specific driver analyses. Fig. 2: Pathway and driver analysis identifies driver genes in the long tail of the driver p -values for coding and non-coding mutations. a Pathway and network methods identify significant coding driver mutations. Driver p -values on protein-coding elements for 250 genes with most significant coding driver p -values; dashed and dotted lines indicate FDR = 0.1 and 0.25, respectively. Dark green bars are PID-C genes, and light green bars are non-PID-C genes. Blue squares below the x -axis indicate COSMIC Cancer Gene (CGC) Census genes. In total, 31 of 87 PID-C genes have coding driver p -values with FDR > 0.1. Several PID-C genes are labeled, including all CGC genes with coding FDR > 0.1. Overlap between PID-C and PID-N genes is indicated with asterisks. Source data are provided as a Source Data file. b Pathway and network methods identify rare non-coding driver mutations. Driver p -values on non-coding elements (promoter, 5′ UTR, and 3′ UTR of gene) for 250 genes with most significant non-coding driver p -values; dashed and dotted lines indicate FDR = 0.1 and 0.25, respectively. Dark yellow bars are PID-N genes, and light yellow bars are non-PID-N genes. Blue squares are as above. In total, 3 ( TERT , HES1 , and TOB1 ) of 93 PID-N genes have non-coding driver p -values with FDR ≤ 0.1, while 90 have FDR > 0.1 . Several PID-N genes are labeled, including PID-N genes with significant in cis gene expression changes (see Fig. 3 ) and all PID-N genes with non-coding FDR > 0.25. Overlap between PID-C and PID-N genes is indicated with asterisks. Source data are provided as a Source Data file. c Statistical significance of overlap between top-ranked genes according to coding driver p -values and PID-C genes with CGC genes. Fisher’s exact test p -values and driver FDR thresholds of 0.1 and 0.25 are highlighted. Green squares indicate overlap between PID-C genes and CGC genes. Source data are provided as a Source Data file. d Statistical significance of overlap of genes ranked by driver p -values on non-coding (promoter, 5′ UTR, 3′ UTR) elements and CGC genes. Driver FDR thresholds of 0.1 and 0.25 are highlighted. Yellow square indicates overlap between PID-N genes and CGC genes. Source data are provided as a Source Data file. Full size image Using non-coding mutations alone, we identify a set of 62 genes using our consensus pathway and network analysis, resulting in fewer genes than our analysis with coding mutations. However, when we performed a joint analysis of coding and non-coding mutations, we found that the much stronger signal in coding mutations dominated the combined signal in coding and non-coding mutations. To increase sensitivity to detect contributions of non-coding mutations, we devised a “non-coding value-added” (NCVA) procedure (Fig. 1 ; Supplementary Fig. 3 ; Non-coding value-added (NCVA) procedure in the Methods section). Our NCVA procedure asks if the coding mutations enhance the discovery of potential non-coding driver genes beyond what is found with only the non-coding mutations. This procedure identified an additional set of 31 genes that, when merged with the 62 genes found with non-coding mutations alone, resulted in a set of 93 pathway-implicated driver genes with non-coding variants (PID-N) (Supplementary Fig. 4 , Consensus results in the Methods section). PID-N genes appear as a robust and biologically relevant set, unbiased by any particular mutational process reflecting a particular carcinogen or DNA damage processes (Supplementary Fig. 5 , Mutational signatures in the Methods section). The 93 PID-N genes (Supplementary Data 3 , Supplementary Fig. 6b ) include 19 previously identified cancer genes according to the COSMIC Cancer Gene Census (CGC) database a significant enrichment over the 3.2 genes expected ( p = 5.3 × 10 −11 ; Fisher’s exact test, Fig. 2b, d ; Supplementary Figs. 7b, c ). Excluding the eight genes with individually significant non-coding elements in the PCAWG Drivers and Functional Interpretation Working Group analysis [16] , 19 genes are both PID-N genes and CGC genes, a significant enrichment over the 3.1 genes expected ( p = 5.3 × 10 −11 ; Fisher’s exact test), suggesting that non-coding mutations may alter genes with recurrent coding or structural variants in some samples. The PID-N genes have significantly higher non-coding gene scores than non-PID-N genes (rank-sum test p = 1.47 × 10 −58 ; median rank 165 of PID-N genes), and 92/93 PID-N genes (except for HIST1H2BO ) improve the scores of their network neighborhoods (28.5 genes expected; p < 10 −6 ; Supplementary Data 10 ). This shows that PID-N genes are not implicated solely by their network neighbors [14] . The vast majority of PID-N genes (90/93, including the 19 CGC genes) are distinct from the PCAWG Drivers and Functional Interpretation Working Group analysis (Fig. 2b ; Supplementary Figs. 8b , 9 ), with only three genes in common: TERT , HES1 , and TOB1 . Of these three, only TERT is recorded as a known cancer gene in the CGC database. Moreover, the 93 PID-N genes are more strongly enriched ( p = 5.3 × 10 −11 ; Fisher’s exact test) for COSMIC CGC genes than the 93 genes with the smallest non-coding driver p -values of promoters, 5′ UTRs, or 3′ UTRs ( p = 4.8 × 10 −3 ; Fisher’s exact test). Thus, our consensus procedure of the pathway and network analyses appreciably augments the significantly mutated elements in the PCAWG Drivers and Functional Interpretation Working Group results [16] . Taken together, the PID-C and PID-N genes contain an additional 121 genes over what was found in the PCAWG Drivers and Functional Interpretation Working Group analysis, including 90 new possible non-coding drivers (Consensus Results in the Methods section). In total, non-coding mutations in PID-N genes cover an additional 151 samples (9.1% of samples) than PID-C genes. We found that most coding mutations in PID-C genes and most non-coding mutations in PID-N genes are clonal (median > 80% for both PID-C and PID-N genes [26] ). In addition, the overwhelming majority of the PID-N genes were distinct from PID-C genes (Supplementary Fig. 4 ) with only five genes in common: CTNNB1 , DDX3X , SF3B1 , TGFBR2 , and TP53 . While this suggests that coding and non-coding driver mutations occur in largely distinct sets of cancer genes, we show below that both types of mutations affect genes underlying many of the same hallmark cancer processes. Impact of non-coding mutations on gene expression Non-coding mutations may act by altering transcription factor-binding sites or other types of regulatory sites. Thus, we evaluated whether non-coding mutations in PID-N genes were associated with in cis expression changes in the same gene. We found that five PID-N genes (FDR < 0.3) showed significant in cis expression correlations out of the 90 that could be tested using RNA-Seq data (Fig. 3 ; Supplementary Fig. 10 ; Supplementary Data 11 – 16 ). In contrast, 34 out of 87 PID-C genes exhibited significant or near-significant in cis expression correlations (FDR < 0.3) (Supplementary Data 17 , 18 ). Fig. 3: Gene expression changes are correlated with mutations in PID-N genes. Evolutionary conservation of genomic elements estimated with PhyloP are shown as gray features. H3 histone lysine 4 tri-methylation sites (H3K4me3) measured in GM12878 HapMap B-lymphocytes cell lines are highlighted in the green track, indicating active promoter regions near transcription start sites [49] . Boxplot center lines show the median, boxplot bounds show the first quartile Q1 and the third quartile Q3, and whiskers show 1.5 (Q3–Q1) below and above Q1 and Q3, respectively. a TP53 promoter. TP53 coding and non-coding genomic loci with zoomed-in view of the TP53 promoter region. TP53 promoter mutations (six mutations in Biliary-AdenoCA, ColoRect-AdenoCA, Kidney-ChRCC, Lung-SCC, Ovary-AdenoCA, and Panc-AdenoCA cancer types) correlate significantly (Wilcoxon rank-sum test p = 0.001, FDR = 0.087) with reduced TP53 gene expression, where FPKM-UQ is upper quartile normalized fragments per kilobase million. Samples with copy-number gains and losses in the TP53 promoter region are annotated in red and blue, respectively. Two of the six TP53 promoter mutations overlap with transcription factor-binding sites (with one mutation matching three motifs). Source data are provided as a Source Data file. b TLE4 promoter. TLE4 coding and non-coding genomic loci with zoomed-in view of TLE4 promoter region. TLE4 promoter mutations in Liver-HCC samples (three mutations) correlate (Wilcoxon rank-sum test p = 0.02, FDR = 0.2) with lower TLE4 gene expression. Samples with copy-number gains and losses annotated in red and blue, respectively. One of the three TLE4 promoter mutations has a transcription factor-binding site for ZNF263 . Source data are provided as a Source Data file. c TCF4 promoter. TCF4 coding and non-coding genomic loci with zoomed-in view of TCF4 promoter region. TCF4 promoter mutations in Lung-SCC samples (three mutations) correlate (Wilcoxon rank-sum test p = 0.03, FDR = 0.27) with lower TCF4 gene expression. Samples with copy-number gains and losses annotated in red and blue, respectively. One of the three TCF4 promoter mutations has a transcription factor-binding site for ZEB1 . Source data are provided as a Source Data file. Full size image Unsurprisingly, the most significant in cis expression correlation for a PID-N gene is the correlation between TERT promoter mutations and increased expression, which we find in 11 Thy-AdenoCA tumors ( p = 1.3 × 10 −10 , FDR = 3.2 × 10 −9 ; Wilcoxon rank-sum test), 11 CNS-Oligo tumors ( p = 6.8 × 10 −3 , FDR = 9.7 × 10 −2 ; Wilcoxon rank-sum test), and 22 CNS-GBM tumors (Wilcoxon rank-sum test p = 2.3 × 10 −2 , FDR = 0.19; Wilcoxon rank-sum test) (Supplementary Fig. 8 ), consistent with previous reports [5] , [6] , [27] . Note that these associations were limited by the unavailability of RNA expression data for some samples with TERT mutations as well as the low-sequencing coverage in promoter regions that limited the detection of TERT promoter mutations. The PCAWG Drivers and Functional Interpretation Working Group investigated the latter issue for two mutation hotspot sites in the TERT promoter, and estimated that 216 mutations in these sites were likely not called [16] , a large underrepresentation relative to the total of 97 samples with TERT promoter mutations (71 samples with expression data) in our analyses. We found significant in cis expression correlations in four other PID-N genes: TP53 , TLE4 , TCF4 , and DUSP22 (Fig. 3 , Supplementary Fig. 10 ). TP53 shows significantly reduced expression ( p = 1.0 × 10 −3 ; FDR = 8.7 × 10 −2 ; Wilcoxon rank-sum test) across six tumors with TP53 promoter mutations from six different tumor types (Fig. 3a ; Supplementary Fig. 10 ). The reduced expression of mutated samples is consistent with TP53 ’s well-known role as a tumor suppressor gene, and links between TP53 promoter methylation and expression have been previously investigated [28] . This expression change was also described in the study by the PCAWG Drivers and Functional Interpretation Working Group [16] . TLE4 shows significantly reduced expression ( p = 1.7 × 10 −2 ; FDR = 0.20; Wilcoxon rank-sum test) in three Liver-HCC tumors with TLE4 promoter mutations (Fig. 3b ; Supplementary Fig. 10 ). TLE4 is a transcriptional co-repressor that binds to several transcription factors [29] , and TLE4 functions as a tumor suppressor gene in acute myeloid lymphoma through its interactions with Wnt signaling [30] . Furthermore, in an acute myeloid lymphoma cell line, TLE4 knockdown increased cell division rates, while forced TLE4 expression induced apoptosis [31] . However, the role of TLE4 in solid tumors is not well understood. TCF4 shows significantly reduced expression ( p = 3.4 × 10 −2 ; FDR = 0.27; Wilcoxon rank-sum test) in three Lung-SCC tumors with TCF4 promoter mutations (Fig. 3c ; Supplementary Fig. 10 ). TCF4 is part of the TCF4/β-catenin complex and encodes a transcription factor that is downstream of the Wnt signaling pathway. Low TCF4 expression has been observed in Lung-SCC tumors [32] . Finally, DUSP22 has significantly reduced expressed ( p = 6.3 × 10 −3 ; FDR = 0.024; Wilcoxon rank-sum test) in five Lung-AdenoCA patients with DUSP22 3′ UTR mutations and significantly over-expressed ( p = 7.8 × 10 −4 ; FDR = 0.075; Wilcoxon rank-sum test) in three Lung-AdenoCA patients with DUSP22 5′ UTR mutations. These UTR mutations were mutually exclusive. DUSP22 encodes a phosphatase signaling protein, and was recently proposed to be a tumor suppressor in lymphoma [33] . While these gene expression correlations provide additional support for a subset of PID-N genes, the variant allele frequency of a mutation and the copy number of the gene are additional covariates for gene expression. We found that these covariates did not play a role in of the correlations that we identified: the majority of mutations in each PID gene were clonal (Supplementary Fig. 11 ) and copy-number changes did not affect the expression correlations for the five PID-N genes described above (Fig. 3 ; Supplementary Fig. 10 ). In addition, the low number of PID-N genes exhibiting associated gene expression changes is explained by the low number of samples with mutations in PID-N genes, the uneven availability of expression data across the tumor types, and decreased sequence coverage in promoter regions [16] . These issues further reduced the number of samples with non-coding mutations and RNA expression, limiting the power of in cis gene expression correlation analysis. Modular organization of coding and non-coding mutations We identified specific protein–protein interaction subnetworks and biological pathways that were altered by coding mutations, non-coding mutations, or a combination of both types of mutations. We found significantly more interactions between PID-C genes that expected by chance using a node-degree preserving permutation test (64 interactions observed vs. 40 interactions expected, p < 10 −6 ), a near-significant number of interactions between PID-N genes (18 vs. 12 expected, p = 6.8 × 10 −2 ), and significantly more interactions between both PID-C and PID-N genes (67 vs. 40 expected, p = 6 × 10 −4 ), demonstrating an interplay between coding and non-coding mutations on physical protein–protein interaction networks (Network annotation in the Methods section). We organized the interacting subnetworks involving PID-C and PID-N genes into five biological processes: core drivers, chromatin organization, cell proliferation, development, and RNA splicing (Fig. 4a ). While the high frequency of molecular interactions between PID-C and PID-N genes is expected since such interactions were used as a signal in pathway and network methods, the organization of these interactions illustrates the relative contributions of coding and non-coding mutations in individual subnetworks. Fig. 4: Pathway and network modules containing PID-C and PID-N genes. a Network of functional interactions between PID-C and PID-N genes. Nodes represent PID-C and PID-N genes and edges show functional interactions from the ReactomeFI network (gray), physical protein–protein interactions from the BioGRID network (blue), or interactions recorded in both networks (purple). Node color indicates PID-C genes (green), PID-N genes (yellow), or both PID-C and PID-N genes (orange); node size is proportional to the score of the gene; and the pie chart diagram in each node represents the relative proportions of coding and non-coding mutations associated with the corresponding gene. Dotted outlines indicate clusters of genes with roles in chromatin organization and cell proliferation, which predominantly contain PID-C genes; development, which includes comparable amounts of PID-C and PID-N genes; and RNA splicing, which contains PID-N genes. A core cluster of genes with many known drivers is also indicated. b Pathway modules containing PID-C and PID-N genes. Each row in the matrix corresponds to a PID-C or PID-N gene, and each column in the matrix corresponds to a pathway module enriched in PID-C and/or PID-N genes (see the Methods section). A filled entry indicates a gene (row) that belongs to one or more pathways (column) colored according to gene membership in PID-C genes (green), PID-N genes (yellow), or both PID-C and PID-N genes (orange). A dark colored entry indicates that a PID-C or PID-N gene belongs to a pathway that is significantly enriched for PID-C or PID-N genes, respectively. A lightly colored entry indicates that a PID-C or PID-N gene belongs to a pathway that is significantly enriched for the union of PID-C and PID-N genes, but not for PID-C or PID-N genes separately. Enrichments are summarized by circles adjacent each pathway module name and PID gene name. Boxed circles indicate that a pathway module contains a pathway that is significantly more enriched for the union of the PID-C and PID-N genes than the PID-C and PID-N results separately. The enriched modules and PID genes are clustered into four biological processes: chromatin, development, proliferation, and RNA splicing as indicated. Full size image We further characterized the molecular pathways enriched among our PID-C and PID-N using the g:Profiler web server [34] (Fig. 4b ; Supplementary Fig. 12 , Supplementary Data 19 – 24 , Pathway annotation in the Methods section). Overall, 63 pathways were enriched for PID-C genes and 13 pathways were enriched for PID-N genes (FDR < 10 −6 ). Since our gene-prioritization methods use pathway databases and interaction networks as prior knowledge, it is not surprising that PID-C and PID-N genes are enriched in multiple molecular pathways. However, the enrichment results provide clues about the modular organization of the pathways and allow us to assess the relative contributions of coding and non-coding mutations in each pathway. We further grouped these molecular pathways into 29 modules using overlaps between annotated pathways recorded in the pathway enrichment map (Supplementary Fig. 12 ). For each enriched module, we examined whether PID-C, PID-N, or both types of genes were responsible for the observed enrichment. This produced a clustering of modules and PID genes into four biological processes: chromatin organization, cell proliferation, development, and RNA splicing (Fig. 4b ). We found that pathways in the chromatin and cell proliferation processes—including chromatin remodeling and organization, histone modification, apoptotic signaling, signal transduction, Ras signaling, and cell growth—were altered primarily by coding mutations in PID-C genes. This is not surprising as these pathways contain many well-known cancer genes, such as TP53 , KRAS , BRAF , cyclin-dependent kinase inhibitors, EGFR , PTEN , and RB1 . At the same time, we found that multiple signaling pathways include significant numbers of both PID-C and PID-N genes, suggesting that non-coding mutations provide an alternative to coding mutations in disrupting these pathways. In particular, the Wnt signaling pathway (FDR = 6.8 × 10 −13 ), which was predominantly targeted by coding mutations, was also targeted by non-coding mutations in several PID-N genes, including TERT (103 mutations), HNF1A/B (24 mutations), TLE4 (32 mutations), TCF4 (93 mutations), and CTNNB1 (17 mutations) (Supplementary Fig. 13a ). The Notch signaling pathway (FDR = 6.8 × 10 −7 ) was associated with comparable numbers of PID-C and PID-N genes, including the PID-N genes JAG1 and MIB1 that encode ligands and the PID-N transcription factors ACL1 , HES1 , and HNF1B (66 non-coding mutations in total) (Supplementary Fig. 13b ). The TGF-β signaling pathway (FDR = 3.2 × 10 −7 ) also contained both PID-C and PID-N genes, including the PID-N genes HES1 , HNF1A/B , HSPA5 , MEF2C , and the genes TGFBR2 and CTNNB1 , which are both PID-C and PID-N genes (214 coding mutations and 166 non-coding mutations). We found that several developmental processes were altered by significant numbers of both PID-C and PID-N genes. Cell fate determination (FDR = 2.0 × 10 −7 ) was predominantly affected by non-coding mutations in the PID-N genes DUSP6 , MEF2C , JAG1 , SOX2 , HES1 , ACL1 , ID2 , SUFU, and KLF4 (total 191 non-coding mutations), but also by coding mutations in PID-C genes BRAF , GATA3 , and NOTCH1/2 . Pathways related to nervous system development (FDR = 5.8 × 10 −8 ) were enriched for the PID-N genes ASCL1 , CTNNB1 , ID2 , SUFU , and TERT that have known roles in cancer [35] , [36] , complementing the PID-C genes NOTCH1 , PTEN , and RHOA that also have known cancer roles. The pattern specification process (FDR = 8.8 × 10 −8 ) was also affected by both coding and non-coding mutations, including the PID-N genes ASCL1 , SUFU , and RELN and the PID-C genes ATM and SMAD4 . In these cases, non-coding mutations complement the coding mutations that disrupt these pathways, covering additional patients. Intriguingly, we find that RNA splicing pathways were affected primarily by non-coding mutations (FDR = 7.6 × 10 −9 ). A total of 17 PID-N genes involved in splicing-related pathways (Supplementary Fig. 13c ), including several heterogeneous nuclear ribonucleoproteins (hnNRP) and serine- and arginine-rich splicing factors (SRSFs). None of these PID-N genes were significantly mutated according to single-element tests used in the PCAWG Drivers and Functional Interpretation Working Group analysis [16] . As we did not find any significant (FDR < 0.1) in cis associations between non-coding mutations and altered expression in splicing-related PID-N genes, we explored potential in trans effects between non-coding mutations in these genes and expression of other genes. We found that non-coding mutations in splicing-related PID-N genes largely recapitulate a recently published association from a TCGA PanCanAtlas analysis [37] between coding mutations in several splicing factors and differential expression of 47 pathways (Fig. 5 ). In particular, we identified three clusters of mutations in RNA splicing genes (C1, C2, and C3; Fig. 5a, b ) using hierarchical clustering of differential expression patterns across these pathways. A highly overlapping set of clusters was found using t -distributed stochastic neighbor embedding (top annotation bar in Fig. 5a ) showing that the clusters were robust to the choice of the clustering method. Further support for robustness of clusters was found via silhouette scores and bootstrapping (Supplementary Fig. 14 ). Each of these clusters contained at least one coding mutation in the splicing genes SF3B1 , FUBP1 , and RBM10 , as reported previously [37] , along with non-coding mutations in splicing-related PID-N genes, demonstrating that both types of mutations resulted in similar gene expression signatures. The joint analysis of coding and non-coding mutations in splicing factors also recovered the two groups of enriched pathways [37] (P1 and P2 in Fig. 5a ; Supplementary Fig. 15 ). One group (P1) is characterized by immune cell signatures and the other group (P2) reflects mostly cell-autonomous gene signatures of cell cycle, DDR, and essential cellular machineries [37] . This similarity between the gene expression signatures for non-coding mutations in several PID-N splicing factors and the signatures previously reported for coding mutations in splicing factor genes [37] supports a functional role for splicing-related PID-N genes in altering similar gene expression programs. Fig. 5: RNA splicing factors are targeted primarily by non-coding mutations and alter expression of similar pathways as coding mutations in splicing factors. a Heatmap of Gene Set Enrichment Analysis (GSEA) Normalized Enrichment Scores (NES). The columns of the matrix indicate non-coding mutations in splicing-related PID-N genes and coding mutations in splicing genes reported in ref. [37] , and the rows of the matrix indicate 47 curated gene sets [37] . Red heatmap entries represent an upregulation of the pathway in the mutated samples with respect to the non-mutated samples, and blue heatmap entries represent a downregulation. The first column annotation indicates mutation cluster membership according to common pathway regulation. The second column annotation indicates whether a mutation is a non-coding mutation in a PID-N gene or a coding mutation, with the third column annotation specifies the aberration type (promoter, 5′ UTR, 3′ UTR, missense, or truncating). The fourth column annotation indicates the cancer type for coding mutations. The mutations cluster into three groups: C1, C2, and C3. The pathways cluster into two groups: P1 and P2, where P1 contains an immune signature gene sets and P2 contains cell-autonomous gene sets. b t-SNE plot of mutated elements. Gene expression signatures for samples with non-coding mutations clusters in splicing-related PID-N genes with gene expression signatures for coding mutations in previously published splicing factors. The shape of each point denotes the mutation cluster assignment (C1, C2, or C3), and the color represents whether the corresponding gene is a PID-N gene with non-coding mutations or a splicing factor gene with coding mutations. Full size image In addition to the above modules, we also found that transcription factors were well represented among both the PID-C and PID-N genes. In total, nine PID-C genes are transcription factors ( ARHGAP35 , ARID2 , FOXA1 , GATA3 , NFE2L2 , SMAD4 , SOX9 , TCF7L2 , TP53 ; FDR = 2.1 × 10 −10 ), while 19 PID-N genes are transcription factors ( ASCL1 , BHLHE40 , ESRRG , HES1 , HNF1A , HNF1B , HOXA10 , HOXB5 , KLF4 , MEF2C , MYC , NFE2 , NR2F1 , SOX2 , SOX4 , TCF4 , TP53 , ZNF521 , ZNF595 ; FDR = 4.1 × 10 −20 ). This observation suggests that non-coding mutations may affect transcriptional regulatory networks. We present an integrative pathway and network analysis that expands the list of genes with possible non-coding driver mutations into the “long tail” of rarely mutated elements that are not significant by single-element analysis. We find that genes harboring both coding or non-coding mutations overlap in pathways and networks; thus, pathway databases and interaction networks serve as useful sources of prior knowledge to implicate additional mutated elements beyond those identified by single-element tests. In total, our integrative pathway and network analysis identified 87 pathway-implicated driver genes with coding variants (PID-C) and 93 pathway-implicated driver genes with non-coding variants (PID-N). Importantly, 90 PID-N genes were not statistically significant (FDR > 0.1) by single-element tests on non-coding mutation data, and these genes are key candidates for future experimental characterization. Among them, we find that promoter mutations in TP53 , TLE4 , and TCF4 are associated with reduced expression of these genes. We find that coding and non-coding driver mutations largely target different genes and make varying contributions to pathways and networks perturbed in cancer. While some cancer pathways are targeted by both coding and non-coding mutations, such as the Wnt and Notch signaling pathways, other pathways appear to be predominantly altered by one class of mutations. In particular, we find non-coding mutations in multiple genes in the RNA splicing pathway, and samples with these mutations exhibit gene expression signatures that are concordant with gene expression changes observed in samples with coding mutations splicing factors SF3B1 , FUBP1 , and RBM10 [37] . Together these results demonstrate that rare non-coding mutations may result in similar perturbations to both common and complementary biological processes. There are several caveats to the results reported in this study. First, there is relatively low power to detect non-coding mutations in the cohort, particularly in cancer types with small numbers of patients. Second, transcriptomic data were available for only a subset of samples, further reducing our ability to validate our predictions using gene expression data. Third, our pathway and network analysis relied on the driver p -values from the PCAWG Drivers and Functional Interpretation Working Group analysis [16] . While this analysis accounts for regional variations in the background mutation rate across the genome, it is possible that these corrections are incomplete. Furthermore, if the uncorrected confounding variables are correlated with gene membership in pathways and subnetworks, then the false positive rates in our analysis may be higher than estimated. All of these factors, plus other unknown confounding variables, make it difficult to assess the false discovery rate of our predictions, particularly for PID-N genes. Further experimental validation of these predictions is necessary to determine the true positives from false positives in our PID gene lists. Because of limited power in individual cancer types, our pathway and network analysis focused on associations found across cancer and tissue types. Thus, we primarily utilized generic, tissue-independent network and pathway information. However, it is well known that gene–gene interactions vary across tissues and that cancer cells rewire signaling and regulatory networks. Future investigations that consider the variable landscape of regulatory and physical interactions across tissues may offer a new perspective on the data. Specifically, each cell type has a different epigenetic wiring and regulatory machinery, and non-coding mutations may target cell type-dependent vulnerabilities. Approaches that incorporate tissue-specific, cancer-specific, or patient-specific gene–gene regulatory information may reveal new classes of drivers unexplored with our current approaches. Our pathway- and network-driven strategies enable us to interpret the coding and non-coding landscape of tumor genomes to discover driver mechanisms in interconnected systems of genes. This approach has multiple benefits. First, by broadening our mutation analysis from single genomic elements to pathways and networks of multiple genes, we identify new components of known cancer pathways that are recurrently altered by both coding and non-coding mutations, and thus likely to be important in cancer. Second, we identify new pathways and subnetworks that would remain unseen in an analysis focusing on coding sequences. Investigation of the coding and non-coding mutations that perturb these pathways and networks will enable more accurate patient-stratification strategies, pathway-focused biomarkers, and therapeutic approaches. Mutation and pathway data We used gene scores derived from the PCAWG Drivers and Functional Interpretation Working Group analysis [16] and combined several pathways and interaction networks for our pathway and network analyses. Here, we use the term “pathway methods” to refer to approaches that utilize sets of related genes for their analysis and use the term “network methods” to refer to approaches that utilize pairwise interactions among genes and/or their products. Somatic mutation data We obtained consensus driver p -values ( syn8494939 ) from the PCAWG Drivers and Functional Interpretation Working Group analysis [16] for coding and non-coding (core promoter, 5′ UTR, 3′ UTR, enhancers) genomic elements for the Pancan-no-skin–melanoma–lymph cohort. We removed driver p -values for several elements ( H3F3A and HIST1H4D coding; LEPROTL1 , TBC1D12 , and WDR74 5′ UTR; and chr6:142705600-142706400 enhancer, which targets ADGRG6 ) that the PCAWG Drivers and Functional Interpretation Working Group analysis had manually examined and discarded. We included enhancers with ≤ 5 gene targets (syn7201027), which covered 89% of enhancers elements from the PCAWG Drivers and Functional Interpretation Working Group analysis [16] . In cases where the PCAWG Drivers and Functional Interpretation Working Group analysis reported multiple p -values for the same genomic element, we used the smallest reported p -value for that element. Derivation of gene scores Pathway databases and gene interaction networks typically record information at the level of individual genes. Thus, we formed coding and non-coding gene scores by combining PCAWG driver p -values across coding and/or non-coding (core promoter, 5′ UTR, 3′ UTR, enhancer) genomic elements as follows. Let p x ( g ) be the driver p -value for element x of gene g from the PCAWG Drivers and Functional Interpretation Working Group analysis [16] . We combined p -values from multiple elements using Fisher’s method, where we selected the minimum p -value min( p promoter ( g ), p 5’UTR ( g )) for overlapping core promoter and 5′ UTR elements on gene g and the minimum p -value p enhancer ( g ) of all enhancers targeting gene g . Using this approach, we defined the following gene scores on coding (GS-C), non-coding, (GS-N), and combined coding and non-coding (GS-CN) genomic elements: 1. GS-C: p C ( g ) = p coding ( g ) 2. GS-N: p N ( g ) = fisher(min( p promoter ( g ), p 5′UTR ( g )), p 3′UTR ( g ), p enhancer ( g )) 3. GS-CN: p CN ( g ) = fisher( p coding (g), min( p promoter ( g ), p 5′UTR ( g )), p 3′UTR ( g ), p enhancer ( g )). Here, \(p = {{{\mathrm{fisher}}}}(p_1, \ldots ,p_k) = - 2\mathop {\sum}\nolimits_{i = 1}^k {{{{\mathrm{ln}}}}} \left( {p_i} \right)\sim \chi _{2k}^2\) , is Fisher’s method for combining p -values, where 2k is the degrees of freedom in the calculation. When the driver p -value for a genomic element was undefined, we omitted that element from the calculation and reduced the number of degrees of freedom. For the pathway and networks methods that analyze individual mutations, we used mutations from the PCAWG MAF ( syn7364923 ) on the same genomic elements as the PCAWG Drivers and Functional Interpretation Working Group analysis, i.e., coding, core promoter, 5′ UTR, 3′ UTR, and enhancer. We removed melanoma and lymphoma samples as well as 69 hypermutated samples with over 30 mutations/MB (syn7894281, syn7814911). We also removed mutations in elements that the PCAWG Drivers and Functional Interpretation Working Group analysis had manually examined and discarded (see above), resulting in lists of mutations used for later assessing biological relevance of our results ( syn8103141 , syn9684700 ). Pathway and network databases Pathway methods used gene sets from six databases: CORUM [38] , GO [39] , InterPro [40] , KEGG [41] , NCI Nature [42] , and Reactome [43] ( syn3164548 , syn11426307 ), where small (<3 genes) and large (>1000 genes) pathways were removed. Network methods used interactions from three interaction networks: the largest connected subnetwork of the ReactomeFI 2015 interaction network [44] ( syn3254781 ) with high-confidence (≥ 0.75 confidence score) interactions, which we treated as undirected; the largest connected subnetwork of the iRefIndex14 interaction network [45] , which we augmented with interactions from the KEGG pathway database [41] ( syn10903761 ). The BioGRID interaction network [46] ( syn3164609 ) was also used to evaluate and annotate results. Individual pathway and network algorithms We applied seven pathway and network methods to the gene scores and mutation data. We used two pathway methods: ActivePathways [19] and a hypergeometric analysis (Vazquez). We also used five network methods: CanIsoNet [20] , Hierarchical HotNet [21] , an induced subnetwork analysis (Reyna and Raphael, in preparation), NBDI [22] , and SSA-ME [23] . 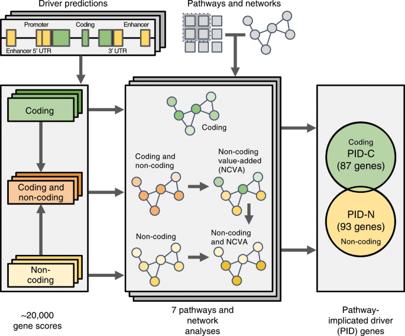Fig. 1: Overview of the pathway and network analysis approach. Coding, non-coding, and combined gene scores were derived for each gene by aggregating driverp-values from the PCAWG driver predictions in individual elements, including annotated coding and non-coding elements (promoter, 5′ UTR, 3′ UTR, and enhancer). These gene scores were input to five network analysis algorithms (CanIsoNet20, Hierarchical HotNet21, an induced subnetwork analysis (Reyna and Raphael, in preparation), NBDI22, and SSA-ME23), which utilize multiple protein–protein interaction networks, and to two pathway analysis algorithms (ActivePathways19and a hypergeometric analysis (Vazquez)), which utilize multiple pathway/gene-set databases. We defined a non-coding value-added (NCVA) procedure to determine genes whose non-coding scores contribute significantly to the results of the combined coding and non-coding analysis, where NCVA results for a method augment its results on non-coding data. We defined a consensus procedure to combine significant pathways and networks identified by these seven algorithms. The 87 pathway-implicated driver genes with coding variants (PID-C) are the set of genes reported by a majority (≥4/7) of methods on the coding data. The 93 pathway-implicated driver genes with non-coding variants (PID-N) are the set of genes reported by a majority of methods on non-coding data or in their NCVA results. Only five genes (CTNNB1,DDX3X,SF3B1,TGFBR2, andTP53) are both PID-C and PID-N genes. Table 1 shows pathway databases and interaction networks used by each method. Table 1 Summary of pathway database and interaction network data for each method. Full size table Using these pathway and network databases, we ran each method on the GS-C, GS-N, and GS-CN gene scores to identify three corresponding lists of genes. Each method evaluated the statistical significance of its results on each data set. Non-coding value-added (NCVA) procedure The GS-CN results leverage both coding and non-coding mutation data, improving the detection of weaker pathway and network signals. We devised a non-coding value-added (NCVA) procedure to separate the coding and non-coding signals in this combined analysis, resulting in a set of NCVA genes for which the non-coding mutation data make a statistically significant contribution to their discovery in the GS-CN results. Specifically, we evaluated the statistical significance of genes in the GS-CN results using a permutation test where the driver p -values for coding elements were fixed and the driver p -values for non-coding elements were permuted. This procedure identified the subset of the GS-CN results that were reported infrequently ( p < 0.1) on permuted data, and thus more likely to be true positives. Each method’s NCVA results were added to that method’s overall set of non-coding results (GS-N). Consensus results for pathway and network methods We defined a consensus set of genes for each set of results: GS-C results, GS-N results, GS-CN results, and GS-N combined with NCVA results, across our seven pathway and network methods. Specifically, we defined a gene to be a consensus gene if it was found by a majority (≥ 4/7) of the pathway and network methods. For our analysis, we focused on the consensus GS-C results, which we call the pathway-implicated driver genes with coding variants (PID-C), and the consensus from the GS-N results combined with NCVA results, which we call the pathway-implicated driver genes with non-coding variants (PID-N). We defined PID-C genes as the 87 genes in the consensus of the GS-C results, and we defined PID-N genes as the 93 genes in the consensus of each method’s GS-N results combined with its NCVA results. We performed several analyses to assess the biological relevance of PID-C and PID-N genes. Identification of mutational signatures of PID genes We performed a permutation-based enrichment test for mutation signatures from PCAWG mutation signatures analysis [47] . We identified the most likely mutation signature for each non-coding mutation in PID-N genes and compared them to randomly chosen non-coding mutations in non-PID-N genes. Improved network neighborhood scores of PID genes To assess the extent to which gene scores on PID genes contribute to their detection by pathway and network methods, we considered the contribution of each PID gene’s score to the score of its network neighborhood in the BioGRID interaction network. For each PID gene g , we used Fisher’s method to combine the gene scores of the first-order network neighbors of g both with and without the score of g itself. In particular, for gene g , let p ( g ) be the gene score for g and N ( g ) be the network neighborhood of g . Then 
    p_N(g)^with = fisher( p(v):v ∈ N( g ) ∪{ g })
 is a score for the network neighborhood of g when including gene g and 
    p_N(g)^without = fisher( p(v):v ∈ N( g ))
 is a score for the network neighborhood of g when excluding gene g . If the network neighborhood of g has a smaller p -value with g than without g , i.e., \(p_{N(g)}^{{{{\mathrm{with}}}}} \, < \, p_{N(g)}^{{{{\mathrm{without}}}}}\) , then gene g improves the score of the network neighborhood, suggesting that the gene score of g plays a role in its detection by pathway and network methods. Alternatively, if the network neighborhood of g has a larger p -value with g than without g , i.e., \(p_{N(g)}^{{{{\mathrm{with}}}}} \, > \, p_{N(g)}^{{{{\mathrm{without}}}}}\) , then gene g worsens the score of the network neighborhood, suggesting that the gene scores of the network neighbors of g are predominantly responsible for the detection of g by pathway and network methods. We performed this test for every PID-C gene with GS-C gene scores and every PID-N gene with GS-N gene scores. We also sampled genes uniformly at random from the network (87 for PID-C genes and 93 for PID-N genes; 10 6 trials) to ascertain whether significantly more PID genes that improved the scores of their network neighborhoods than expected by chance. Expression analysis of PID genes We evaluated whether mutation status of each PID gene was correlated with RNA expression. We used PCAWG-3 gene expression data ( syn5553991 ), which was averaged from TopHat2 and STAR-based alignments, with FPKM-UQ normalization. Tumor type and copy-number aberrations are known to be covariates for gene expression, so we conditioned on tumor types and annotated copy-number aberrations. We used the following procedure to assess expression correlations on individual tumor types. We only considered cases with at least three mutated samples and three non-mutated samples to restrict our analysis to cases with sufficient statistical power. For each PID-C gene or each non-coding element in a PID-N gene, we partitioned the samples with expression data into a set A of samples with mutation(s) in the element and a set B of samples without mutations in the element. We performed the Wilcoxon rank-sum test for the expression of the gene in sets A and B and performed the Benjamini–Hochberg correction on each coding or non-coding element to provide FDRs. We used the following procedure to assess expression correlations across tumor types. We only considered cases with at least one mutated sample and one non-mutated sample to restrict our analysis to cases with sufficient statistical power. For each PID-C gene and each non-coding element in a PID-N gene, we partitioned the samples with expression data into sets A c of samples in cohort c with mutation(s) in the element and sets B c of samples in cohort c without mutations in the element. We converted the expression values into z -scores using the expression from non-mutated samples in cohort c , and we computed the Wilcoxon rank-sum test on the expression of the gene in sets from A = ⋃ c ∊ C A c and B = ⋃ c ∊ C B c , where C is the set of all cohorts containing samples with mutation(s) in the element. We then performed the Benjamini–Hochberg correction on each coding or non-coding element to provide FDRs. Network annotation of PID genes We performed a permutation test to evaluate the statistical significance of the number of interactions in the BioGRID high-confidence interaction network between PID-C genes, the number of interactions between PID-N genes, and the number of interactions between PID-C and PID-N genes, i.e., when a PID-C gene interacts with a PID-N gene. To compute the permutation p -value, we sampled random networks uniformly at random from the collection of networks with the same degree sequence as the BioGRID network. We found connected subnetworks of 46 PID-C genes (31 genes expected, p = 9 × 10 −4 ) and 16 PID-N genes (10 genes expected, p = 6.1 × 10 −2 ) in the high-confidence BioGRID [48] protein–protein interaction (PPI) network. The union of the PID-C and PID-N genes formed a larger connected subnetwork of 73 genes (Fig. 4a ). These connected subnetworks were significantly larger than expected by chance according to this permutation test (57 genes expected, p = 2.2 × 10 −3 ). Furthermore, we observed statistically significant numbers of protein–protein interactions between PID-C and PID-N genes (67 interactions observed vs. 45 expected, p = 6 × 10 −4 ), suggesting that the associated mutations may target an overlapping set of underlying pathways. The PID-C genes were connected by significantly more interactions than expected (64 vs. 40 expected, p < 10 −4 ), and the PID-N genes were interconnected at a sub-significant level (18 vs 12 expected, p = 6.8 × 10 −2 ). Thus, certain pathways are affected by either coding or non-coding mutations, but some pathways are affected by a complement of both coding and non-coding mutations. Pathway annotation of PID genes Using g:Profiler [34] , we performed a pathway enrichment analysis for PID genes and 12,061 gene sets representing GO biological processes and Reactome pathways. We used the Benjamini–Hochberg correction to control the FDR of the results. Characterization of PID genes in RNA splicing GSEA enrichment analysis was performed with the default parameters using the curated pathway gene lists [37] for samples harboring non-synonymous coding mutations in five genes ( FUBP1 , RBM10 , SF3B1 , SRSF2 , and U2AF1 ) with confirmed on-target splicing deregulation. Due to limited number of samples with RNA-seq data in individual tumor types, we restricted our analysis to missense mutations in SF3B1 , truncating mutations in RBM10 , and truncating mutations in FUBP1 for tumor types contained at least three samples with these classes of mutations. Each tumor type containing such mutations was considered separately [37] . We performed the same GSEA analysis for non-coding mutations in 17 PID-N genes that were annotated as involved in RNA splicing. Due to limited number of samples from individual tumor types containing mutations in these genes (often there was only one per tumor type), we performed GSEA analysis jointly on all tumor types containing mutations in an individual PID-N gene, restricting the non-mutated group to samples from the same tumor types as the mutant samples. The GSEA Normalized Enrichment Scores (NES) were clustered using hierarchical complete linkage clustering on the Euclidean distance between the NES scores. Separately, we computed a 2D projection of NES scores using t-Distributed Stochastic Neighbor Embedding (t-SNE). 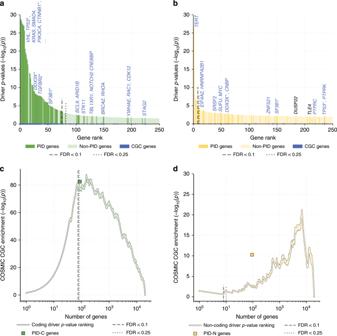Fig. 2: Pathway and driver analysis identifies driver genes in the long tail of the driverp-values for coding and non-coding mutations. aPathway and network methods identify significant coding driver mutations. Driverp-values on protein-coding elements for 250 genes with most significant coding driverp-values; dashed and dotted lines indicate FDR = 0.1 and 0.25, respectively. Dark green bars are PID-C genes, and light green bars are non-PID-C genes. Blue squares below thex-axis indicate COSMIC Cancer Gene (CGC) Census genes. In total, 31 of 87 PID-C genes have coding driverp-values with FDR > 0.1. Several PID-C genes are labeled, including all CGC genes with coding FDR > 0.1. Overlap between PID-C and PID-N genes is indicated with asterisks. Source data are provided as a Source Data file.bPathway and network methods identify rare non-coding driver mutations. Driverp-values on non-coding elements (promoter, 5′ UTR, and 3′ UTR of gene) for 250 genes with most significant non-coding driverp-values; dashed and dotted lines indicate FDR = 0.1 and 0.25, respectively. Dark yellow bars are PID-N genes, and light yellow bars are non-PID-N genes. Blue squares are as above. In total, 3 (TERT,HES1, andTOB1) of 93 PID-N genes have non-coding driverp-values with FDR ≤ 0.1, while 90 have FDR > 0.1 . Several PID-N genes are labeled, including PID-N genes with significant in cis gene expression changes (see Fig.3) and all PID-N genes with non-coding FDR > 0.25. Overlap between PID-C and PID-N genes is indicated with asterisks. Source data are provided as a Source Data file.cStatistical significance of overlap between top-ranked genes according to coding driverp-values and PID-C genes with CGC genes. Fisher’s exact testp-values and driver FDR thresholds of 0.1 and 0.25 are highlighted. Green squares indicate overlap between PID-C genes and CGC genes. Source data are provided as a Source Data file.dStatistical significance of overlap of genes ranked by driverp-values on non-coding (promoter, 5′ UTR, 3′ UTR) elements and CGC genes. Driver FDR thresholds of 0.1 and 0.25 are highlighted. Yellow square indicates overlap between PID-N genes and CGC genes. Source data are provided as a Source Data file. 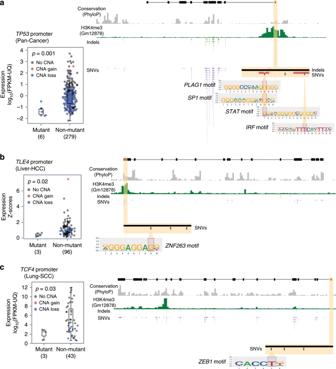Fig. 3: Gene expression changes are correlated with mutations in PID-N genes. Evolutionary conservation of genomic elements estimated with PhyloP are shown as gray features. H3 histone lysine 4 tri-methylation sites (H3K4me3) measured in GM12878 HapMap B-lymphocytes cell lines are highlighted in the green track, indicating active promoter regions near transcription start sites49. Boxplot center lines show the median, boxplot bounds show the first quartile Q1 and the third quartile Q3, and whiskers show 1.5 (Q3–Q1) below and above Q1 and Q3, respectively.aTP53 promoter.TP53coding and non-coding genomic loci with zoomed-in view of theTP53promoter region.TP53promoter mutations (six mutations in Biliary-AdenoCA, ColoRect-AdenoCA, Kidney-ChRCC, Lung-SCC, Ovary-AdenoCA, and Panc-AdenoCA cancer types) correlate significantly (Wilcoxon rank-sum testp= 0.001, FDR = 0.087) with reducedTP53gene expression, where FPKM-UQ is upper quartile normalized fragments per kilobase million. Samples with copy-number gains and losses in theTP53promoter region are annotated in red and blue, respectively. Two of the sixTP53promoter mutations overlap with transcription factor-binding sites (with one mutation matching three motifs). Source data are provided as a Source Data file.bTLE4promoter.TLE4coding and non-coding genomic loci with zoomed-in view ofTLE4promoter region.TLE4promoter mutations in Liver-HCC samples (three mutations) correlate (Wilcoxon rank-sum testp= 0.02, FDR = 0.2) with lowerTLE4gene expression. Samples with copy-number gains and losses annotated in red and blue, respectively. One of the threeTLE4promoter mutations has a transcription factor-binding site forZNF263. Source data are provided as a Source Data file.cTCF4promoter.TCF4coding and non-coding genomic loci with zoomed-in view ofTCF4promoter region.TCF4promoter mutations in Lung-SCC samples (three mutations) correlate (Wilcoxon rank-sum testp= 0.03, FDR = 0.27) with lowerTCF4gene expression. Samples with copy-number gains and losses annotated in red and blue, respectively. One of the threeTCF4promoter mutations has a transcription factor-binding site forZEB1. Source data are provided as a Source Data file. 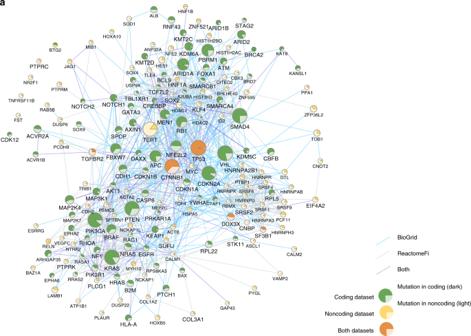Fig. 4: Pathway and network modules containing PID-C and PID-N genes. aNetwork of functional interactions between PID-C and PID-N genes. Nodes represent PID-C and PID-N genes and edges show functional interactions from the ReactomeFI network (gray), physical protein–protein interactions from the BioGRID network (blue), or interactions recorded in both networks (purple). Node color indicates PID-C genes (green), PID-N genes (yellow), or both PID-C and PID-N genes (orange); node size is proportional to the score of the gene; and the pie chart diagram in each node represents the relative proportions of coding and non-coding mutations associated with the corresponding gene. Dotted outlines indicate clusters of genes with roles in chromatin organization and cell proliferation, which predominantly contain PID-C genes; development, which includes comparable amounts of PID-C and PID-N genes; and RNA splicing, which contains PID-N genes. A core cluster of genes with many known drivers is also indicated.bPathway modules containing PID-C and PID-N genes. Each row in the matrix corresponds to a PID-C or PID-N gene, and each column in the matrix corresponds to a pathway module enriched in PID-C and/or PID-N genes (see the Methods section). A filled entry indicates a gene (row) that belongs to one or more pathways (column) colored according to gene membership in PID-C genes (green), PID-N genes (yellow), or both PID-C and PID-N genes (orange). A dark colored entry indicates that a PID-C or PID-N gene belongs to a pathway that is significantly enriched for PID-C or PID-N genes, respectively. A lightly colored entry indicates that a PID-C or PID-N gene belongs to a pathway that is significantly enriched for the union of PID-C and PID-N genes, but not for PID-C or PID-N genes separately. Enrichments are summarized by circles adjacent each pathway module name and PID gene name. Boxed circles indicate that a pathway module contains a pathway that is significantly more enriched for the union of the PID-C and PID-N genes than the PID-C and PID-N results separately. The enriched modules and PID genes are clustered into four biological processes: chromatin, development, proliferation, and RNA splicing as indicated. 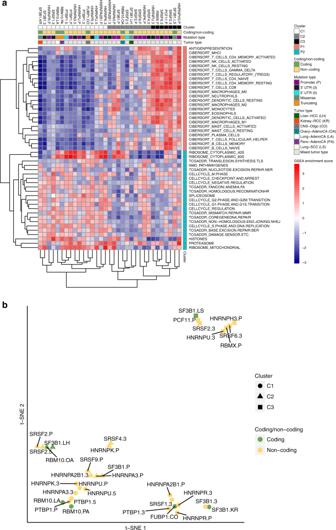Fig. 5: RNA splicing factors are targeted primarily by non-coding mutations and alter expression of similar pathways as coding mutations in splicing factors. aHeatmap of Gene Set Enrichment Analysis (GSEA) Normalized Enrichment Scores (NES). The columns of the matrix indicate non-coding mutations in splicing-related PID-N genes and coding mutations in splicing genes reported in ref.37, and the rows of the matrix indicate 47 curated gene sets37. Red heatmap entries represent an upregulation of the pathway in the mutated samples with respect to the non-mutated samples, and blue heatmap entries represent a downregulation. The first column annotation indicates mutation cluster membership according to common pathway regulation. The second column annotation indicates whether a mutation is a non-coding mutation in a PID-N gene or a coding mutation, with the third column annotation specifies the aberration type (promoter, 5′ UTR, 3′ UTR, missense, or truncating). The fourth column annotation indicates the cancer type for coding mutations. The mutations cluster into three groups: C1, C2, and C3. The pathways cluster into two groups: P1 and P2, where P1 contains an immune signature gene sets and P2 contains cell-autonomous gene sets.bt-SNE plot of mutated elements. Gene expression signatures for samples with non-coding mutations clusters in splicing-related PID-N genes with gene expression signatures for coding mutations in previously published splicing factors. The shape of each point denotes the mutation cluster assignment (C1, C2, or C3), and the color represents whether the corresponding gene is a PID-N gene with non-coding mutations or a splicing factor gene with coding mutations. Ethical review Sequencing of human subjects' tissue was performed by ICGC and TCGA consortium members under approval of local Institutional Review Boards (IRBs). Informed consent was obtained from all human participants. All data were deidentified for this study, and data access for participating researchers was obtained through data access agreements between local institutions, the ICGC Data Access Compliance Office (DACO), and the NIH dbGaP.